Two-way traffic of glycoside hydrolase family 18 processive chitinases on crystalline chitin Processivity refers to the ability of synthesizing, modifying and degrading enzymes to catalyse multiple successive cycles of reaction with polymeric substrates without disengaging from the substrates. Since biomass polysaccharides, such as chitin and cellulose, often form recalcitrant crystalline regions, their degradation is highly dependent on the processivity of degrading enzymes. Here we employ high-speed atomic force microscopy to directly visualize the movement of two processive glycoside hydrolase family 18 chitinases (ChiA and ChiB) from the chitinolytic bacterium Serratia marcescens on crystalline β-chitin. The half-life of processive movement and the velocity of ChiA are larger than those of ChiB, suggesting that asymmetric subsite architecture determines both the direction and the magnitude of processive degradation of crystalline polysaccharides. The directions of processive movements of ChiA and ChiB are observed to be opposite. The molecular mechanism of the two-way traffic is discussed, including a comparison with the processive cellobiohydrolases of the cellulolytic system. Polymers are ubiquitous in living systems: for example, DNA and RNA are essential for storage and transcription of genetic information, proteins have multiple structural and functional roles in cells, and polysaccharides are used for energy storage, exoskeleton formation in animals and structural fibres in plants. Therefore, polymer synthesis and degradation are crucial processes in living organisms. The enzymes involved exhibit processivity, which is defined as the ability to perform multiple successive rounds of catalysis without detachment from the substrate, and the degree of processivity is a key characteristic of such enzymes [1] . In the degradation process of recalcitrant crystalline polysaccharides, such as cellulose (a 1,4-β-linked polymer of D -glucose) and chitin (a 1,4-β-linked polymer of N -acetyl- D -glucosamine GlcNAc), by the corresponding glycanases (cellulases and chitinases), high processivity is one of the most important factors influencing the efficiency of degradation [2] , [3] . These substrates are typically insoluble; however, the hydrolytic products are water-soluble dimers or oligomers. Adsorption of the enzymes on the surface of the substrate is the initial step, and then the polysaccharide chain is loaded into the active site tunnel or cleft of the catalytic module, the glycosidic bond is cleaved by hydrolysis, the reaction product is released and the catalytic module slides along the polymer substrate to the next cleavage site. The reactions are heterogeneous, and the enzymes acting at a solid–liquid interface need to overcome the decrystallization energy during the process [4] , [5] , [6] . Although vast numbers of glycanases are predicted to work processively, it has been difficult to evaluate processivity by means of biochemical experiments, and therefore the structure–function relationship of processive glycanases is poorly understood. In the present study, we visualize the movement of single molecules of two processive glycoside hydrolase (GH) family 18 chitinases (ChiA and ChiB) from the Enterobacteria Serratia marcescens on crystalline β-chitin isolated from tubeworm Lamellibrachia satsuma , using high-speed atomic force microscopy (HS-AFM). Since the molecular chains of chitin are packed with parallel orientation in the crystal [7] , the processive movement of the enzyme molecules can be directly visualized using the procedure described in our previous reports on HS-AFM studies of processive cellulases from the cellulolytic ascomycete Trichoderma reesei [8] , [9] , [10] . There was an advantage of using chitinases rather than cellulases for the present work: the chitinolytic bacterium S. marcescens [11] produces only two extracellular processive chitinases, ChiA and ChiB, and these two enzymes comprise one of the best studied pairs of processive enzymes acting on cellulose/chitin [12] . Both enzymes carry GH family 18 catalytic modules, although ChiA carries the N-terminal chitin-binding domain (ChBD), while ChiB carries the C-terminal CBM family 5 ChBD [12] , [13] . These two enzymes have been predicted to have different directions of hydrolysis, based on transmission electron microscopic observation of the residual crystalline chitin after hydrolysis [14] . Using the HS-AFM technology, we have succeeded in visualizing the catalytic processive movements of ChiA and ChiB, and obtained the first direct evidence that the active enzymes move in opposite directions on crystalline chitin. HS-AFM observations of S. marcescens ChiA A suspension of β-chitin purified from L. satsuma ( Fig. 1a,b ) was dropped on a highly oriented pyrolytic graphite (HOPG) disc and subjected to HS-AFM as illustrated schematically in Fig. 1c . Chitin, a polymer of GlcNAc, is packed into microcrystals that contain more than 1,000 chains, and since one hydrophobic surface of these crystals faces the HOPG disc, chitinases presumably bind to the opposing hydrophobic surface ( Fig. 1c ). In the HS-AFM observation, enzymes can be added during the observation period, and their real-time movement on the same microfibrils can be followed before and after the addition of another enzyme. As shown in Fig. 2a and Supplementary Movie 1 , ChiA moved unidirectionally from right to left (in the images) on the surface of crystalline β-chitin. To confirm that each round bulge represents a single enzyme molecule, its size was compared with that of a simulated AFM image of ChiA created from the crystal structure of this enzyme. As shown in Fig. 2b , the size of the observed and simulated images matched well in both the x–y dimensions and height, suggesting each bulge represents a single ChiA molecule. However, since the density of enzyme molecules moving on crystalline chitin was high and thereby it was difficult to distinguish the individual molecules among the frames, we constructed a kymograph of sliced images and tracked the position of every molecule from Supplementary Movie 1 ( Fig. 2c ). The bright diagonal lines in the kymograph indicate movements of individual ChiA molecules on the substrate surface. In the crystalline chitin used in this study, called β-chitin, the chitin chains are packed in parallel orientation and therefore the processive enzyme molecules all move in the same direction, as indicated by the fact that the slopes are all in the same direction in the kymograph. Moreover, there is only a limited number of stopping molecules (that is, vertical lines in the kymograph), indicating that almost all molecules are moving. 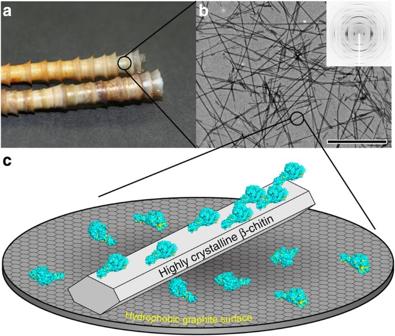Figure 1: Schematic representations of the HS-AFM experiments. (a) TubewormL. satsumaused in the present study. (b) Transmission electron microscopy pictures of highly crystalline β-chitin from tubeworm. Inset shows synchrotron X-ray fibre diffraction diagrams of the preparation. Scale bar indicates 2 μm. (c) Schematic presentation ofS. marcescenschitinase A (ChiA) degrading crystalline β-chitin fromL. satsumafor HS-AFM observation. Figure 1: Schematic representations of the HS-AFM experiments. ( a ) Tubeworm L. satsuma used in the present study. ( b ) Transmission electron microscopy pictures of highly crystalline β-chitin from tubeworm. Inset shows synchrotron X-ray fibre diffraction diagrams of the preparation. Scale bar indicates 2 μm. ( c ) Schematic presentation of S. marcescens chitinase A (ChiA) degrading crystalline β-chitin from L. satsuma for HS-AFM observation. 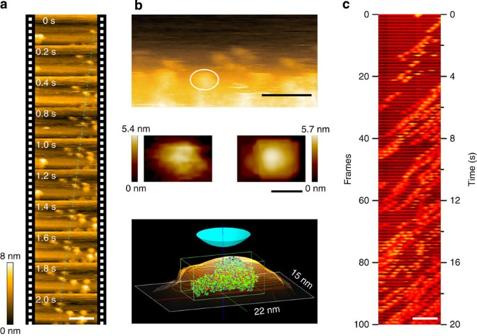Figure 2: The HS-AFM observation of ChiA on crystalline chitin. (a) Real-time observation of crystalline chitin incubated with 1 μM ChiA by means of HS-AFM. The time interval between images is 0.2 s (150 × 75 nm2, 150 × 75 pixels, scan velocity: 112.5 μm s−1). These images are taken fromSupplementary Movie 1with an application of background compensation for a forward tilt of original image as shown inb. Scale bar indicates 60 nm. (b) Comparison of actual and simulated AFM images of ChiA molecules. The left middle image is a height analysis of the molecule circled in white in the top picture. The right middle image is the simulated image of a ChiA molecule created using SPM simulator (Advanced Algorithm & Systems Co.) as shown in the bottom picture. Scale bars for top and middle pictures are 40 and 10 nm, respectively. (c) Kymographic analysis of ChiA movement on crystalline chitin. The kymograph was analysed using a routine developed the in Igor Pro software, as described in Methods. Scale bar indicates 60 nm. Full size image Figure 2: The HS-AFM observation of ChiA on crystalline chitin. ( a ) Real-time observation of crystalline chitin incubated with 1 μM ChiA by means of HS-AFM. The time interval between images is 0.2 s (150 × 75 nm 2 , 150 × 75 pixels, scan velocity: 112.5 μm s −1 ). These images are taken from Supplementary Movie 1 with an application of background compensation for a forward tilt of original image as shown in b . Scale bar indicates 60 nm. ( b ) Comparison of actual and simulated AFM images of ChiA molecules. The left middle image is a height analysis of the molecule circled in white in the top picture. The right middle image is the simulated image of a ChiA molecule created using SPM simulator (Advanced Algorithm & Systems Co.) as shown in the bottom picture. Scale bars for top and middle pictures are 40 and 10 nm, respectively. ( c ) Kymographic analysis of ChiA movement on crystalline chitin. The kymograph was analysed using a routine developed the in Igor Pro software, as described in Methods. Scale bar indicates 60 nm. Full size image Comparison of moving velocity and processivity of chitinases As shown in Fig. 3a and Supplementary Movie 2 , the movement of ChiB was also unidirectional. However, as shown in Fig. 3b versus Fig. 2c , fewer molecules of ChiB than ChiA were observed at the same concentration. Since only productively bound enzyme molecules are visualized in the HS-AFM analysis, the lower frequency of appearance of ChiB might be because of lower affinity of ChiB for the substrate [15] . The diagonal lines in the kymograph indicate that all the molecules are productively bound and are moving linearly on the surface of the substrate. 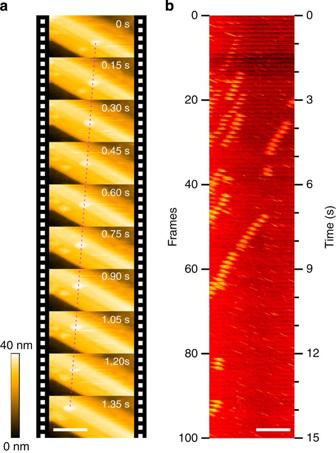Figure 3: HS-AFM images of crystalline β-chitin degradation by ChiB. (a) Real-time observation of crystalline chitin incubated with 1 μM ChiB by means of HS-AFM. The time interval between images is 0.15 s (200 × 100 nm2, 150 × 75 pixels, scan velocity: 200 μm s−1). Scale bar indicates 80 nm. (b) Kymographic analysis of ChiB movement. These images are taken fromSupplementary Movie 2. Scale bar indicates 80 nm. Figure 3: HS-AFM images of crystalline β-chitin degradation by ChiB. ( a ) Real-time observation of crystalline chitin incubated with 1 μM ChiB by means of HS-AFM. The time interval between images is 0.15 s (200 × 100 nm 2 , 150 × 75 pixels, scan velocity: 200 μm s −1 ). Scale bar indicates 80 nm. ( b ) Kymographic analysis of ChiB movement. These images are taken from Supplementary Movie 2 . Scale bar indicates 80 nm. Full size image The movements of S. marcescens ChiA and ChiB were further analysed in order to estimate their kinetic characteristics. 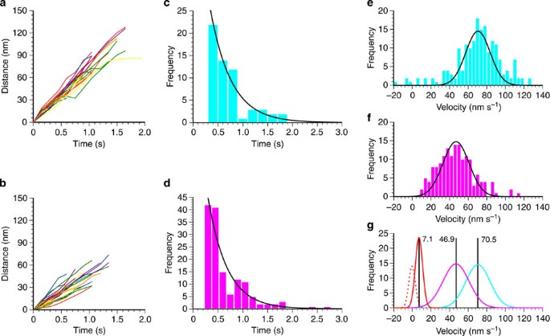Figure 4: Statistical analyses of processive movements of ChiA and ChiB. (a,b) Time courses of distance from the initial position for ChiA and ChiB molecules, respectively. Different colours indicate different molecules observed in HS-AFM images. (c,d) Histograms of the duration for the processive movement of ChiA and ChiB, respectively. (e,f) Velocity distributions of the linear movement of ChiA (e,n=181) and ChiB (f,n=155) on crystalline chitin, respectively. The mobility of each molecule was analysed using a routine developed in the Igor Pro software, as described in Methods. (g) Comparison of the velocity distribution of ChiA (cyan), ChiB (magenta) andTrCel7A (red). The velocity distribution ofTrCel7A is taken from our previous report8. Figure 4a,b shows the time courses of moving distance of ChiA and ChiB created from the kymographs, respectively. Although the velocity of movement both varied from molecule to molecule, ChiA shows longer and faster means of movement than that of ChiB. The histogram of distribution for the duration time of the processive movement was then created ( Fig. 4c,d ), and the half-life of processive movements ( τ )±s.d. was estimated to be 0.293±0.036 and 0.267±0.035 s for ChiA and ChiB, respectively. Figure 4e,f shows the histograms of movement velocities of the two enzymes, and the normality of the distribution of movement velocity was assessed by the normal probability plot as shown in Supplementary Fig. 1A (ChiA) and Supplementary Fig. 1B (ChiB). Although the plots deviate at low and high velocities, both had high correlation coefficients ( R 2 ) of 0.96 and 0.98 for ChiA and ChiB, respectively, indicating that the velocity distribution is approximately normal for both enzymes. The mean velocities±s.d. were 70.5±25.2 and 46.9±19.8 nm s −1 for ChiA ( n =181) and ChiB ( n =155), respectively. From these values—that is, τ and velocities—the half-life of processivity for ChiA was estimated to be 21 reactions, whereas that of ChiB was estimated to be 13 considering the length of the N , N ′-diacetylchitobiose repeating unit is 1.0 nm in crystalline β-chitin [7] . Figure 4: Statistical analyses of processive movements of ChiA and ChiB. ( a , b ) Time courses of distance from the initial position for ChiA and ChiB molecules, respectively. Different colours indicate different molecules observed in HS-AFM images. ( c , d ) Histograms of the duration for the processive movement of ChiA and ChiB, respectively. ( e , f ) Velocity distributions of the linear movement of ChiA (e, n =181) and ChiB (f, n =155) on crystalline chitin, respectively. The mobility of each molecule was analysed using a routine developed in the Igor Pro software, as described in Methods. ( g ) Comparison of the velocity distribution of ChiA (cyan), ChiB (magenta) and Tr Cel7A (red). The velocity distribution of Tr Cel7A is taken from our previous report [8] . Full size image Different orientations of movement of ChiA and ChiB In the present work, we directly confirmed that ChiA and ChiB have opposite moving directions ( Fig. 5 and Supplementary Movies 3 and 4 ). When ChiB alone was initially observed, the enzyme molecules moved from top left to bottom right as shown in Supplementary Movie 3 and magenta lines in Fig. 5a , while after ChiA was added, movement from bottom right to top left was observed (cyan lines). Although we could not distinguish ChiA and ChiB visualized with HS-AFM, the movement of opposite direction appeared only after the two kinds of enzyme were mixed, as shown in Supplementary Movie 4 . Although the final concentrations of ChiA and ChiB were the same (1 μM), ChiA molecules was observed much often than ChiB, as already noted, presumably because of stronger interaction of ChiA with the substrate, as compared with ChiB, owing to the presence of more hydrophobic aromatic amino acids forming a more extended substrate-binding cleft at the subsites [12] , [13] , [16] as described in the Discussion section. 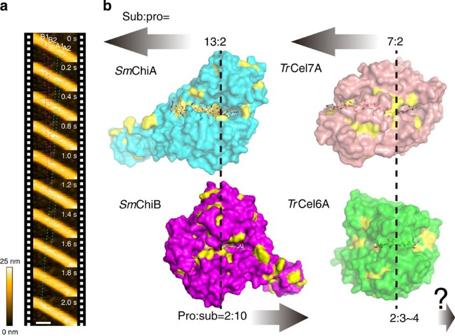Figure 5: Opposite direction of processive movements of chitinases on crystalline chitin. (a) HS-AFM images of crystalline β-chitin degradation by ChiA and ChiB. The time interval between images is 0.2 s (200 × 120 nm2, 100 × 76 pixels, scan velocity: 152 μm s−1). These images are taken fromSupplementary Movie 3. Cyan and magenta lines indicate the movements of ChiA and ChiB, respectively. The processive direction was decided when ChiB alone was incubated with the substrate, as described in the Methods section. Scale bar indicates 60 nm. (b) Structural comparison ofSmChiA (PDB: 1K9T),SmChiB (PDB: 1UR9 (ref.32)),TrCel7A (PDB: 8CEL (ref.33)) andTrCel6A (1QK2 (ref.34)). Dashed lines indicate the location at which hydrolysis occurs. The ratio Sub:Pro or Pro:Sub shows the ratio of the numbers of binding sites for substrate (Sub) and product (Pro). Figure 5: Opposite direction of processive movements of chitinases on crystalline chitin. ( a ) HS-AFM images of crystalline β-chitin degradation by ChiA and ChiB. The time interval between images is 0.2 s (200 × 120 nm 2 , 100 × 76 pixels, scan velocity: 152 μm s −1 ). These images are taken from Supplementary Movie 3 . Cyan and magenta lines indicate the movements of ChiA and ChiB, respectively. The processive direction was decided when ChiB alone was incubated with the substrate, as described in the Methods section. Scale bar indicates 60 nm. ( b ) Structural comparison of Sm ChiA (PDB: 1K9T), Sm ChiB (PDB: 1UR9 (ref. 32 )), Tr Cel7A (PDB: 8CEL (ref. 33 )) and Tr Cel6A (1QK2 (ref. 34 )). Dashed lines indicate the location at which hydrolysis occurs. The ratio Sub:Pro or Pro:Sub shows the ratio of the numbers of binding sites for substrate (Sub) and product (Pro). Full size image Crystalline polysaccharides often form the skeletal parts of living organisms, such as crystalline cellulose in plant cell walls and crystalline chitin in the Crustacea. These structural polysaccharides are physically strong and are not easily degraded, unlike deposited sugars such as starch. However, they are available in large amounts in nature, and so the possibility of utilizing them to make chemicals and fuels (biorefining) is extremely attractive. In developing technologies for biomass utilization, a detailed understanding of the processivity of crystalline polysaccharide-degrading glycanases is critical. The processivity of glycanases has been studied by means of biochemical experiments so far [17] ; however, this is problematic because of the great difficulty in distinguishing between multiple exo-type reactions catalysed by plural enzyme molecules and a processive reaction catalysed by a single molecule. In our previous studies of cellulases, we used HS-AFM to visualize processive movements of individual cellobiohydrolase (CBH) molecules on crystalline cellulose [8] , [9] , [10] . In the present study, we applied this technique to chitin-degrading enzymes, and we have succeeded in visualizing the unidirectional movement of S. marcescens ChiA and ChiB on crystalline β-chitin. During our previous HS-AFM observations of processive cellulases, we realized that enzyme molecules bound non-productively, such as those of GH family 7 endoglucanase I from T. reesei ( Tr Cel7B), which lacks hydrolytic activity towards crystalline cellulose, are hardly visualized [18] . This is because molecules without hydrolytic activity would quickly dissociate from the substrate and therefore would not be clearly visualized in more than one frame. However, the inability of the technique to observe non-productive enzyme molecules can be turned to advantage, in that visualization of only productively bound molecules allows HS-AFM to be used for analysis of the processivity of glycanases that degrade crystalline polysaccharides. Although the direction of movement also cannot be determined from HS-AFM observation, previous biochemical results [13] , morphological observations of β-chitin after hydrolysis [14] , [19] and the molecular structure of the enzymes [20] , [21] all clearly indicate that ChiA moves from the reducing end to the non-reducing end, and ChiB moves to opposite direction of ChiA on the chitin polymer chain [22] . Although processivity is difficult to estimate from biochemical experiments [17] , processivity values of 9.1 and 3.4 have been reported for S. marcescens ChiA and ChiB, respectively, on chitosan (a partially deacetylated derivative of chitin) as a substrate [16] , [22] . The values on chitin estimated from the present HS-AFM data are ~2.3 (ChiA) and 3.7 (ChiB) times greater than those reported for chitosan hydrolysis. GH family 18 chitinases such as ChiA and ChiB employ a substrate-assisted hydrolytic mechanism, and the acetamide residue of chitin is indispensable; therefore, the high processivity values we estimated may simply reflect the smaller extent of deacetylation in the substrate using in the present study. On the other hand, the tendency that the processivity of ChiA is about twice that of ChiB is common, and this may reflect the fact that the substrate-binding site in ChiA is longer than that of ChiB, as discussed below [12] , [19] . Our observed velocities are similar to the velocities of hydrolysis of hexa- N -acetylchitohexaose (soluble hexamer of GlcNAc) previously reported by Horn et al . [15] , for which the initial rates of ChiA and ChiB were 46 and 35 s −1 , respectively, suggesting that the degradation of crystalline chitin resembles the hydrolysis of soluble oligosaccharide. The velocity distributions of ChiA and ChiB were then compared with that of Tr Cel7A, a processive cellulase ( Fig. 4g ). In the case of the cellulase [8] , the velocity of movement was estimated to be 7.1 s −1 ; therefore, it may appear that ChiA moves 10 times faster than Tr Cel7A. However, we cannot simply compare the velocities of the chitinases and cellulase because the crystalline substrates are different. In particular, crystalline β-chitin used in this study contains water molecules in the crystal [7] , which may strongly influence the activities of glycan hydrolases. Assuming that each processive movement involves catalysis, the moving velocities suggest that a single catalytic process takes 0.014 and 0.021 s for ChiA and ChiB, respectively, whereas Tr Cel7A needs 0.14 s (ref. 8 ). Considering that the frame rate of HS-AFM used for the observation was 0.15–0.20 s, each frame includes ~10 catalytic cycles for chitinases, while several catalyses were in one frame for Tr Cel7A. This is one possible reason why we rarely observed standstill of the chitinases, whereas apparent stop of the movement of Tr Cel7A during the processive motion was observed, as shown by the dotted histogram line in Fig. 4g . It is also possible that the ‘cleft-type’ active site causes faster off-rate of chitinases from the substrate than processive cellulase with ‘tunnel-type’ catalytic domain. As already mentioned, the domain architectures of ChiA and ChiB are opposite—that is, ChiA has an N-terminal fibronectin type III-like ChBD, whereas ChiB has a C-terminal CBM family 5 ChBD with an extended catalytic subsite cleft—and it has been suggested that this difference of molecular structure would result in opposite directions of hydrolysis of chitin chains [12] , [14] , [15] , [19] , [22] , [23] . The molecular architectures of S. marcescens chitinases (ChiA and ChiB) and T. reesei cellulases ( Tr Cel7A and Tr Cel6A) are compared in Fig. 5b . The enzymes that move from the reducing end to the non-reducing end ( Sm ChiA and Tr Cel7A) bind the substrate at negative subsites (−13 to −1 in Sm ChiA and −7 to −1 in Tr Cel7A) and bind the product at positive subsites (+1 and +2), whereas the enzyme that move from the non-reducing end to the reducing end have the opposite arrangement—that is, the substrate is bound at subsites +1 to +10 in Sm ChiB and subsites +1 to +3~4 in Tr Cel6A—while the product is bound at subsites −1 and −2. However, when these molecules are aligned based on the catalytic centre (between subsites −1 and +1), there is an apparent difference between the enzymes that were seen to move using HS-AFM ( Sm ChiA, Sm ChiB and Tr Cel7A) and the enzyme that did not appear to move ( Tr Cel6A) [8] . Specifically, the enzymes that were seen to move had a substrate-binding site that was much longer than the product-binding site, irrespective of where the sites were located (positive or negative side). In other words, ‘asymmetric architecture’ of the substrate-binding and product-binding sites seems to be the key to the linear movement of such glycanases in HS-AFM observations, as had already been predicted from biochemical and structural comparisons of ChiA and ChiB [20] , [21] , [22] . In a previous study on cellulase, a tunnel-shaped catalytic domain was considered to be essential for processive action, based on a comparison of fungal GH family 6 and 7 CBHs and endoglucanases [24] . Indeed, we could not observe the movement of Tr Cel7B, which has a cleft-type subsite with a similar catalytic domain to Tr Cel7A. However, as discussed above and shown in Fig. 5b , both ChiA and ChiB moved processively on crystalline chitin in the present experiments, even though they have cleft-type but not tunnel-type subsites. Thus, a tunnel-shaped catalytic domain does not seem to be required for processive movement. Considering that Tr Cel7B has similar asymmetric subsite architecture to that of Tr Cel7A, asymmetricity alone does not seem to be sufficient for processivity in the degradation of crystalline polysaccharides. Rather, we suggest that the presence of a long substrate-binding site (more than 10 GlcNAc units) formed by the ChBD is one of the key factors to high processivity of chitinases. In our recent study about fungal GH family 7 CBHs using HS-AFM, there are several loops covering subsites and these may interfere with release of the substrate from the catalytic domain, resulting in slower movement of Tr Cel7A than similar CBHs from basidiomycete Phanerochaete chrysosporium ( Pc Cel7C and Pc Cel7D), showing trade-off relationship between hydrolytic velocity and processivity [18] . Moreover, Payne et al . [25] recently demonstrated that the processivity of GH family 7 CBHs directly relates to the ligand binding free energy calculated by molecular dynamics, indicating that higher affinity to the substrate chain causes higher processivity of these enzymes. Unlike the results of GH family 7 CBHs, both processivity and moving velocity of ChiA are higher than those of ChiB in the present observation using HS-AFM. There is a major difference between the cellulases and chitinases—that is, processivity is mainly driven by catalytic domain in GH family 7 CBHs—while extended structure including CBM decides the processivity and moving direction in GH family 18 chitinases (ChiA and ChiB). Considering that a single mutation of one aromatic amino acid lowers the processivity and increases hydrolytic activity in ChiA as demonstrated in the former biochemical study [22] , the balance between velocity and processivity is ‘fine-tuned’ by controlling the affinity with the substrates [15] . There is an interesting difference between bacterial crystalline chitinolytic and fungal crystalline cellulolytic systems. Thus, S. marcescens utilizes two highly processive enzymes moving in different directions, which may have evolved by the addition of a short linker and CBM-like domain. On the other hand, T. reesei has high- and low-processivity enzymes, which have a flexible long linker and a small nonspecific CBM. Preparation of crystalline β-chitin and enzymes Satsuma tubeworms ( L. satsuma ) were collected from the sea off Kagoshima Bay at a depth of about 100 m using a remotely operated vehicle, Hyper-Dolphin (JAMSTEC, Japan). The bodies of the tubeworms were removed by washing the tube with water, and the tubes were kept in deionized water in a refrigerator. The never-dried tubes kept in deionized water were cut into ~3 cm lengths and were then deproteinized according to the method described previously [26] . After overnight immersion in 1 N NaOH solutions at room temperature, they were treated with 0.3% NaClO 2 solutions buffered at pH 4.9 in 0.1 M acetate buffer at 70 °C for 3 h [7] , [26] . Recombinant chitinase A (ChiA) and chitinase B (ChiB) from the chitinolytic bacteria S. marcescens were heterologously expressed in Escherichia coli DH5α cells harbouring plasmids pNCA112 carrying the cloned chiA gene [27] and pMCB7 carrying the cloned chiB gene [28] for ChiA and ChiB, respectively. The crude proteins obtained after sonication of the cells were collected by ammonium sulfate precipitation (80% saturation) and were dissolved in 1.0 mM sodium phosphate buffer (pH 6) and purified by hydroxyapatite column (ϕ3.0 × 7.0 cm) according to the previous report [29] . The chitinase fractions were applied to chitin affinity column previously equilibrated with 20 mM phosphate buffer (pH 6) containing 0.5 M NaCl. After washing with three column volumes of the same buffer and three column volumes of 20 mM sodium acetate buffer (pH 5.5), chitinase was eluted with 20 mM acetic acid. Peak fractions containing chitinase were collected and used as purified enzyme samples as described in the previous report [27] . High-speed AFM observations High-speed AFM observations were carried out using a laboratory-built customized HS-AFM apparatus and operated with tapping mode [30] . We used a small cantilever (BL-AC10EGS-A2; Olympus Corporation), which is 10 μm long, 2 μm wide and 90 nm thick with a spring constant of ~0.1 N m −1 . Its resonant frequency and quality factor in an aqueous solution are ~600 kHz and ~2, respectively. For AFM imaging, the free oscillation amplitude was ~2 nm and the set-point amplitude was ~90% of the free oscillation amplitude. On the basis of this imaging condition, the tapping force estimated was less than 30 pN [31] . An amorphous carbon tip with the length of ~1 μm was grown on the original tip by electron beam deposition and then the tip apex was sharpened by plasma etching under argon gas (~4 nm in radius). Typical imaging rates used for this study were 0.2 or 0.15 s per frame. For the high-speed AFM observations, 2 μl of crystalline chitin suspension in water (0.2 %) was dropped on a freshly cleaved HOPG substrate, which was rinsed three times with 18 μl of 50 mM MES buffer, pH 6, after incubation for 5 min [8] , [9] . Crystalline chitin on the HOPG substrate was initially observed without enzyme in 70 μl of the same buffer, followed by the addition of an enzyme solution at a final concentration of 1.0 μM. At least three independent chitin microfibrils were observed to estimate the velocity and processivity of chitinases. Chitin microfibrils with a length more than 1 μm were observed for estimation of the processivity of ChiA and ChiB. Construction of kymograph In order to analyse the movements of chitinase molecules along crystalline chitin fibrils, kymographs were constructed using a laboratory-developed AFM image viewer based on Igor Pro (Ver. 6.22, WaveMetrics Inc.). First, we manually drew a straight line along a chitin fibril on the initial image to specify the direction of the fibril, as shown in Supplementary Fig. 2A . Then the image was clipped to leave a rectangular area with a preset width in pixels along the line. The clipped image was rotated so that the longitudinal axis was in a horizontal direction ( Supplementary Fig. 2B ). The successive images were then aligned vertically as shown in Supplementary Fig. 2C . In the resulting kymograph, the linear movements of molecules are readily visualized as bright spots moving along diagonal lines. Tracking analysis using a kymograph For statistical analysis of the velocities of individual chitinase molecules linearly moving on crystalline chitin, semi-automatic tracking of a molecule on the kymograph was carried out using the following procedures. First, we manually selected a molecule on the initial frame on the kymograph and the position of the centre of mass within the selected area (region of interest, ROI) was calculated ( Supplementary Fig. 3A ). The image in the ROI was used as a reference image. Second, we selected the same molecule on the last frame, and the position of the centre of mass was again calculated within the ROI. Then a line was drawn connecting the centres of mass in the first and last frames. Assuming that the molecule moves continuously with a constant velocity, the molecular positions are expected to lie on the line, as indicated by asterisks on Supplementary Fig. 3B . Then, for the second frame the ROI was two-dimensionally swept on a pixel-to-pixel basis around the expected position of the target. The range of pixel shift was normally set to ±15 pixels in both directions. The two-dimensional (2D) correlation coefficient r to the reference image (initial frame) was calculated for each position of the ROI. The 2D correlation coefficient r is defined as follows: where, I mn and R mn are pixel intensities at point ( m , n ) in the analysed image and the reference image, respectively. and are the mean values of the intensity matrices I and R , respectively. In the present case, the analysed image and the reference image correspond to the second and the first images, respectively. The ROI position in the analysed image giving the maximum value of the 2D correlation coefficient was decided. Finally, the position of the centre of mass in the ROI was calculated. The above procedures were repeated for all subsequent frames, including the last frame ( Supplementary Fig. 3C ). Half-life of processive movement ( τ ) was calculated by the curve-fitting of the distribution of duration time to exponential decay (equation 2) as follows: where t is duration time, a 0 is intercept of y axis and τ is half-life of processive movement. The coefficients and s.d. was estimated using the regression-curve-fitting function of the Igor Pro software. How to cite this article: Igarashi, K. et al . Two-way traffic of glycoside hydrolase family 18 processive chitinases on crystalline chitin. Nat. Commun. 5:3975 doi: 10.1038/ncomms4975 (2014).